Two-stroke scooters are a dominant source of air pollution in many cities Fossil fuel-powered vehicles emit significant particulate matter, for example, black carbon and primary organic aerosol, and produce secondary organic aerosol. Here we quantify secondary organic aerosol production from two-stroke scooters. Cars and trucks, particularly diesel vehicles, are thought to be the main vehicular pollution sources. This needs re-thinking, as we show that elevated particulate matter levels can be a consequence of ‘asymmetric pollution’ from two-stroke scooters, vehicles that constitute a small fraction of the fleet, but can dominate urban vehicular pollution through organic aerosol and aromatic emission factors up to thousands of times higher than from other vehicle classes. Further, we demonstrate that oxidation processes producing secondary organic aerosol from vehicle exhaust also form potentially toxic ‘reactive oxygen species’. Particulate matter (PM) damages health [1] and affects climate [2] . Road vehicles are a significant source of PM, particularly in urban areas. A number of recent studies have shown that a large fraction, possibly the largest, of vehicular PM is secondary organic aerosol (SOA) produced via atmospheric oxidation of precursor gases in the exhaust [3] , [4] , [5] . Thus, understanding vehicular air pollution requires an assessment of SOA formation from different vehicle types. Two-stroke (2S) scooters (powered two-wheeled vehicles with engine displacement ≤50 cm 3 ) are popular globally, particularly in Asia, Africa and Southern Europe. 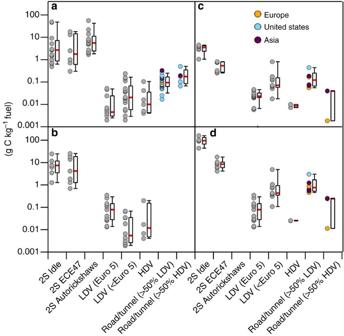Figure 1: Emission factors from scooters and other vehicles. EFs plotted as box-and-whiskers (median line, red; 25th and 75th percentile, box; 10th and 90th percentile, whiskers) of (a) POA, (b) aged OA (POA+SOA formation), (c) benzene and (d) light aromatics (benzene, toluene and C2–C4 alkylated benzenes). Points shown next to the box-and-whiskers are the individual data points, coloured depending on measurement region for ambient data. 2S scooters (this study,n=3) were run in idle or during driving cycles (ECE47). Data on the other vehicles shown are from the literature (Supplementary Table 3) for light-duty and heavy-duty vehicles (LDVs and HDVs). LDVs data are further divided between vehicles meeting Euro 5 and those not meeting Euro 5, labelled <Euro 5 in parenthesis. Ambient data are split according to a contribution of HDVs to the data of higher than or lower than 50%. Note that many of the higher ambient values are from older vehicle studies (Supplementary Table 3). Despite being high emitters of primary PM [6] , [7] , regulations for scooters are generally less stringent than for other vehicles, for example, in Europe having reached Euro 5/V (a fifth tranche of regulations), for passenger cars and trucks, versus only Euro 2 for scooters (see Supplementary Table 1 and ref. 8 ). Accordingly, a scientific report to the European Commission suggests that scooters will emit more volatile organic compounds (VOCs) than all other vehicles combined in Europe by 2020 (ref. 9 ). Furthermore, high PM levels and toxic aromatic hydrocarbons, important SOA precursors [10] , have been observed in many cities, especially in Asia [11] . Globally, organic aerosol (OA) dominates PM, with SOA accounting for the largest fraction [4] . Here we show that 2S scooters emit significant amounts of primary organic aerosol (POA), aromatic VOCs and also produce significant SOA. We use the term ‘asymmetric polluter’ to describe these vehicles as their emission factors (EFs) and evidence from air quality measurements before and after bans on scooters in Asian cities suggest they may dominate vehicular pollution despite their relatively small numbers. Chemical analysis of the emissions shows that SOA is mainly produced via photo-oxidation of aromatic VOCs, present in gasoline, from the exhaust. This shows that the known issue of incomplete fuel combustion during the 2S cycle is also responsible for SOA formation. Finally, we present the first online measurements of aged exhaust showing that SOA formation also produces reactive oxygen species (ROS) with potentially detrimental effects on our lungs. Emission Factors We investigated POA emissions and SOA formation from 2S scooters and their potential health effects. The oxidation of VOCs in 2S scooter emissions produces significant SOA (g carbon (C) kg −1 fuel), with total OA on average 2.9 and 2.4 times higher than POA after aging for idling and driving 2S scooters, respectively ( Fig. 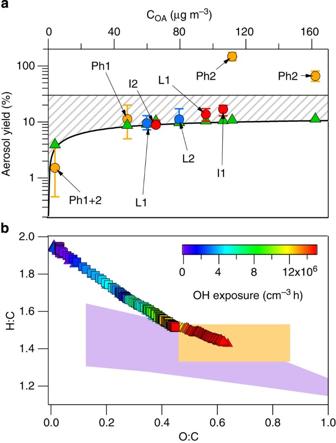Figure 2: Contribution of aromatic oxidation to two-stroke scooter secondary aerosol formation. (a) Apparent SOA mass yields,yapparent(equation (1)), as a function of suspended OA concentration (COA). Error bars show the sensitivity ofyapparentto the chamber wall-loss factor, ±one s.d.yapparentfor a Euro 1 and two Euro 2 2S scooters are shown in red, blue and orange, respectively. Ph 1 and Ph 2 are the first and second phases of the ECE47 driving cycle, I and L refer to idling and simulated low power, respectively. A predicted yield, concentration-weighted, for the mixture of all aromatics (Supplementary Note 1), is given in green triangles. The shaded region denotes the range between maximum (low NOX) and minimum (high NOX) SOA yields form-xylene, a major aromatic constituent of gasoline. (b) Elemental ratios of OA emissions for the Euro 1 (squares) and a Euro 2 (triangles) scooter as a function of photochemical age. Elemental ratios observed for xylene13and ambient31SOA are shown, orange and purple, respectively. 1 , and Supplementary Table 2 ). In addition, substantial toxic aromatic emissions (up to ~\n40% of emitted VOC volume for the scooters of this study) of benzene, toluene and C2–C4 alkylated benzenes, which are recognized SOA precursors [10] , [12] , are present in the exhaust. Among the aromatics, benzene is of particular concern due to its carcinogenicity. Levels in the raw 2S scooter exhaust were as high as 300,000 μg m −3 or 146 p.p.m. (v) from idling. The EU annual mean limit for the protection of human health is 5 μg m −3 (ref. 13 ), while the US National Institute for Occupational Safety and Health recommends that workers wear special breathing equipment when exposed to benzene at levels exceeding 1 p.p.m. for 15 min. Waiting in traffic behind a 2S scooter, for example, at junctions and while the scooter is idling, may therefore be highly deleterious to health. Figure 1: Emission factors from scooters and other vehicles. EFs plotted as box-and-whiskers (median line, red; 25th and 75th percentile, box; 10th and 90th percentile, whiskers) of ( a ) POA, ( b ) aged OA (POA+SOA formation), ( c ) benzene and ( d ) light aromatics (benzene, toluene and C2–C4 alkylated benzenes). Points shown next to the box-and-whiskers are the individual data points, coloured depending on measurement region for ambient data. 2S scooters (this study, n =3) were run in idle or during driving cycles (ECE47). 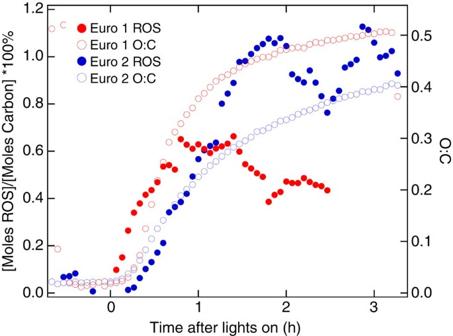Figure 3: Reactive oxygen species in two-stroke scooter emissions. The percentage of water soluble reactive oxygen species (ROS) and elemental O:C ratios of organic aerosol as a function of time after lights on in the smog chamber from Euro 1 (red) and Euro 2 (blue) 2S scooter exhaust emissions. ROS concentration measured in moles hydrogen peroxide equivalents is normalized to the molar organic carbon concentration per m3inside the smog chamber to give a percentage. Data on the other vehicles shown are from the literature ( Supplementary Table 3 ) for light-duty and heavy-duty vehicles (LDVs and HDVs). LDVs data are further divided between vehicles meeting Euro 5 and those not meeting Euro 5, labelled <Euro 5 in parenthesis. Ambient data are split according to a contribution of HDVs to the data of higher than or lower than 50%. Note that many of the higher ambient values are from older vehicle studies ( Supplementary Table 3 ). Full size image Secondary organic aerosol yields The contribution of the aromatics to SOA formation was estimated by calculating an apparent aerosol yield, y apparent , assuming all SOA comes from aromatic precursors: where C SOA is the SOA produced (μg m −3 ) for a given mass change in aromatic i (Δ i , i=benzene, toluene or C2–C4 alkylated benzenes). Apparent yields closely match average concentration-weighted literature aromatic SOA yields [10] ( Fig. 2a , Supplementary Note 1 ) for idling, complete ECE47 driving cycles and ECE47 phase one (Ph1), indicating that most SOA is from aromatic precursors ( Fig. 2a ). SOA from ECE47 phase two (Ph2) alone is underestimated by equation (1), suggesting SOA production from unidentified compounds, emitted by the hot engine. Note that the total emission during a full cycle is dominated by Ph1, that is, by cold engine emissions. Furthermore, a ‘Van Krevelen diagram’ illustrates the aging of 2S scooter emissions, from oxygen to carbon (O:C)~\n0 to O:C~\n0.6. This elemental composition is consistent with that of previously observed SOA from aromatic precursors [14] ( Fig. 2b ). We therefore conclude that SOA formation from 2S scooter emissions is likely from the oxidation of aromatics, in contrast to diesel SOA, which is predominantly from other precursors [15] . Figure 2: Contribution of aromatic oxidation to two-stroke scooter secondary aerosol formation. ( a ) Apparent SOA mass yields, y apparent (equation (1)), as a function of suspended OA concentration ( C OA ). Error bars show the sensitivity of y apparent to the chamber wall-loss factor, ±one s.d. y apparent for a Euro 1 and two Euro 2 2S scooters are shown in red, blue and orange, respectively. Ph 1 and Ph 2 are the first and second phases of the ECE47 driving cycle, I and L refer to idling and simulated low power, respectively. A predicted yield, concentration-weighted, for the mixture of all aromatics ( Supplementary Note 1 ), is given in green triangles. The shaded region denotes the range between maximum (low NO X ) and minimum (high NO X ) SOA yields for m -xylene, a major aromatic constituent of gasoline. ( b ) Elemental ratios of OA emissions for the Euro 1 (squares) and a Euro 2 (triangles) scooter as a function of photochemical age. Elemental ratios observed for xylene [13] and ambient [31] SOA are shown, orange and purple, respectively. Full size image Comparison to other vehicle types and ambient data Figure 1 also shows laboratory and ambient measurements of POA, light aromatic and benzene EFs from passenger cars and trucks ( Supplementary Table 3 ). Ambient data are from roadside/tunnel measurements in the US, EU and Asia, and are split according to the fraction of light-duty and heavy-duty vehicles (LDVs and HDVs, respectively) at the measurement site. Note that the general trend is for lower EFs in newer studies, consistent with improvements in emission controls. Also shown are data from Indian in-use 2S autorickshaws for comparison to the European scooters of this study. Caution is required in such a comparison; however, although similar (both have 2S engines), these are a different vehicle class and were furthermore tested during a different driving cycle. In general, ambient EFs from Asian vehicles are in the same range as European and US vehicles, while emissions from in-use 2S rickshaws are slightly higher than from the European scooters of this study. POA emissions from 2S scooters are on average around 20 (maximum 2,780) times higher than ambient (light-duty dominant) values, and aged OA emissions on an average 53–771 times higher than laboratory studies on other vehicle types. It should be noted that absolute aerosol concentrations can influence EFs: higher measurement concentrations would lead to higher EFs [15] . SOA formation is most significant from idling scooter emissions, while smaller at higher engine loads. However, POA emissions are higher under the latter conditions, and the aggregate POA+SOA emission at high load is comparable with that from idling. Reactive oxygen species We also examined the health implications of the 2S scooter SOA (other than those from the mass increase) using online measurements of particle-bound, water soluble reactive oxygen species (ROS) [16] , which are linked to negative health effects [17] . ROS are undetectable in POA, but accounts for 0.5–1% carbon in the aged OA, suggesting that PM emissions initially become increasingly toxic with aging ( Fig. 3 ). Increasing ROS is consistent with the increased O:C ratio of the aerosol and in line with a previous study showing increased oxidative potential with aging for 2S scooter emissions, albeit at aerosol and oxidant loadings much higher than under ambient conditions [18] . After 1–2 h of irradiation, ROS stabilizes or decreases, as reported previously for organic peroxides, likely due to decomposition processes [19] , [20] . Figure 3: Reactive oxygen species in two-stroke scooter emissions. The percentage of water soluble reactive oxygen species (ROS) and elemental O:C ratios of organic aerosol as a function of time after lights on in the smog chamber from Euro 1 (red) and Euro 2 (blue) 2S scooter exhaust emissions. ROS concentration measured in moles hydrogen peroxide equivalents is normalized to the molar organic carbon concentration per m 3 inside the smog chamber to give a percentage. Full size image There are likely several reasons for these relatively large OA and aromatic emissions from 2S scooters. First, 2S engines, unlike four-stroke (4S), require addition of lubricant oils to the fuel, some of which is emitted in the exhaust. Second, during the 2S engine cycle some of the fresh fuel/air mixture passes directly through the engine [21] , increasing VOC emissions, which may explain the high SOA formation. Third, scooters generally utilize ‘rich combustion’ (low-air/fuel ratio), improving drivability while producing higher CO, VOC and PM emissions (but lower NO X ). Accordingly, the VOC emissions measured here, in particular aromatics as found in raw gasoline, are also on average 124 and 11 times higher from idling and driving 2S scooters, respectively, compared with those from other vehicles. Finally, scooter after-treatment systems are inherently inefficient due to their relatively small size and longer light-off times. Precise estimation of a relative contribution to vehicular PM and aromatics from 2S scooters is difficult, since vehicle regulations vary by country. Another complication arises from the possibility of large contributions to OA from a small number of super-polluting vehicles (of all types). However, many scooters will likely fall into this super-polluting category, especially as a considerable number of scooters are in operation in some regions without any form of emissions control (note that all scooters presented in this study are equipped with two-way oxidation catalysts, which reduce emissions of carbon monoxide and VOCs) and because emissions may be further exacerbated by poor maintenance and tampering, rife for scooters [22] . Furthermore, ambient data in Fig. 1 likely include a number of such super-polluting vehicles. Therefore, our results suggest that 2S scooters are ‘asymmetric polluters’ of OA and aromatics compared with other vehicles. Using the average 2S scooter EF (ECE47 driving cycle) in Fig. 1 suggests that 2S scooters contribute to around 60% of roadside POA in Bangkok, where they account for 10% of fuel consumption ( Fig. 4 ). In a more extreme case (comparing the 75th percentile for scooters and 25th percentile for ambient light-duty dominated), 2S scooters would contribute over 96% to roadside POA. Note that these values are based on the European scooters of this study. As Fig. 1 shows, emissions from some in-use Asian 2S vehicles may be higher, by a factor of three. Since other Asian vehicles are not expected to be more polluting based on Fig. 1 , higher emissions from in-use Asian 2S vehicles would strengthen our conclusion that 2S scooters dominate urban pollution in the region. 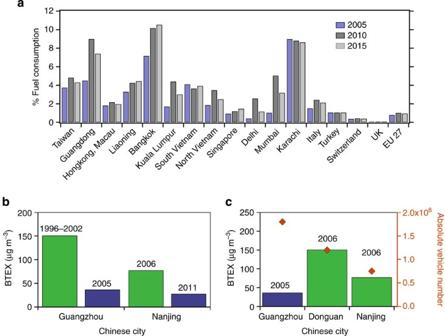Figure 4: Ambient and model data on two-stroke scooters. (a) Share of total fuel consumption by 2S scooters in 2005, 2010 and 2015 from the Greenhouse gas Air pollution Interactions and Synergies, GAINS, model31. (b) Roadside benzene, toluene, ethyl-benzene and xylene (BTEX) before (green) and after (blue) banning/restricting 2S scooters in two Chinese cities (c) Roadside BTEX and number of all vehicles in three Chinese cities, before (green) and after (blue) banning/restricting 2S scooters. Figure 4: Ambient and model data on two-stroke scooters. ( a ) Share of total fuel consumption by 2S scooters in 2005, 2010 and 2015 from the Greenhouse gas Air pollution Interactions and Synergies, GAINS, model [31] . ( b ) Roadside benzene, toluene, ethyl-benzene and xylene (BTEX) before (green) and after (blue) banning/restricting 2S scooters in two Chinese cities ( c ) Roadside BTEX and number of all vehicles in three Chinese cities, before (green) and after (blue) banning/restricting 2S scooters. Full size image Estimation of contributions to aged OA is more difficult as vehicular SOA has not been systematically quantified under ambient conditions. However, smog chamber measurements suggest average-aged OA contributions to ambient vehicular PM of 85% (comparing with LDVs meeting Euro 5) or 98% (comparing with LDVs meeting less than Euro 5) from 2S scooters. Meanwhile, in the EU, 2S scooters consume only 1% of vehicle fuel, Fig. 4 . Even with these low numbers, scooters may be the major source of some of the vehicle-related pollutants, especially in Southern Europe, and our data suggest that reducing the numbers of these vehicles would cost-effectively mitigate vehicle OA and aromatic emissions, given the alternatives available (electric and 4S). In this regard China has taken the lead, banning or restricting scooters in many cities since the late 1990s [23] , leading to large decreases in the traffic-related aromatic emissions in some Chinese cities ( Fig. 4b ). Strikingly, roadside aromatics are now higher in Dongguan, where scooters are not banned, than 60 km away in Guangzhou, even though the traffic volume is much higher in Guangzhou ( Fig. 4c ). This result is statistically significant: year-to-year benzene, toluene, ethyl-benzene and xylene concentrations in Guangzhou were 229 μg m −3 in 1996, 244 μg m −3 in 1999, 290 μg m −3 in 2000 and 150 μg m −3 in 2002, average 228±68 versus 37 μg m −3 after the scooter ban in 2005, for example. Benzene, toluene, ethyl-benzene and xylene concentrations for Guangzhou and other cities reported in the literature are given in Supplementary Table 4 . Our data suggest that 2S scooters are a significant, and in many cities the largest, source of vehicular PM and toxic SOA and aromatic hydrocarbons, despite being a relatively small fraction of the total fleet. Therefore, given the alternative technologies available, restrictions on 2S scooters, already implemented in China, could improve air quality in many cities around the globe. Measurement campaigns We combine results from two measurement campaigns where 2S scooter exhaust was injected through a heated inlet into smog chambers [3] , [24] , [25] to produce SOA via photochemistry. During the first study, an in-use Euro 1 (E1) and a new Euro 2 (E2a) 2S scooter were run in idle or simulated low power. During the second campaign, emissions from a different Euro 2 2S scooter (E2b) were sampled during ECE47 driving cycles [26] . 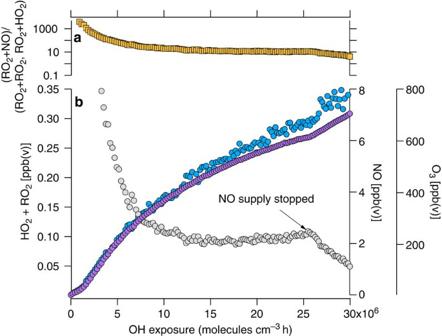Figure 5: Estimation of NOXregime. (a) Calculated branching ratio between nitrate and peroxide reactions (orange squares) in the smog chamber during aging of emissions from an idling 2S scooter and (b) measured concentrations of ozone (O3) (purple circles) and nitrogen monoxide (NO) (grey circles) as well as calculated peroxy radical (HO2+RO2) (blue circles) concentrations. Supplementary Table 5 provides specifications of these vehicles. European (exhaust) emission standards are shown in Supplementary Table 1 . Average OH concentrations were ~\n5 × 10 6 cm −3 . OH concentrations were determined from the decay of a nine times deuterated butanol (butanol-D9, 98% Aldrich) tracer as measured using a quadrupole proton transfer reaction mass spectrometer (idling 2S scooters) or proton transfer reaction time-of-flight mass spectrometer (Ionicon Analytik, driving cycle 2S scooters), see also ref. 27 . Estimation of the NO X regime during experiments Experiments were under ‘high NO X ’ conditions, which we define as the chemical regime where the main reactions of peroxy radicals (RO 2 ) are with NO rather than other peroxy radicals (self-reaction, or reaction with hydroperoxy radicals). An estimate of the ratio of the RO-forming reactions (RO 2 +NO) versus peroxide-forming reactions(RO 2 +RO 2 , RO 2 +HO 2 ) is possible for experiments conducted on idling scooters at the Paul Scherrer Institute chamber, instrumentation for which includes a NO X monitor equipped with a ‘blue light converter’ (ensuring NO X is truly measured as NO 2 +NO). Figure 5b shows the measured concentrations of NO and O 3 , from an experiment conducted on 22 November 2010. This experiment was typical, with an initial VOC:NO X ratio of around 50 and continuous addition of NO during photochemical aging. Figure 5: Estimation of NO X regime. ( a ) Calculated branching ratio between nitrate and peroxide reactions (orange squares) in the smog chamber during aging of emissions from an idling 2S scooter and ( b ) measured concentrations of ozone (O 3 ) (purple circles) and nitrogen monoxide (NO) (grey circles) as well as calculated peroxy radical (HO 2 +RO 2 ) (blue circles) concentrations. Full size image The concentration of NO as a function of time t is given by: Where j NO2 is the photolysis rate of NO 2 in the smog chamber (0.01 s −1 ) and k 1 (1.8 × 10 −14 cm 3 molecule −1 s −1 ) and k 2 (7.7 × 10 −14 cm 3 molecule −1 s −1 ) are the reaction rate constants for NO with O 3 and peroxides (CH 3 O 2 ) at 298 K, respectively. Assuming a steady state of NO (only an approximation, Fig. 5 indicates this point is not reached until around 15 h of OH exposure (at OH=10 6 molecules cm −3 )), equation (2) can be written: Equation (3) suggests NO concentrations at least an order of magnitude higher than RO 2 +HO 2 (for example, 14 times higher at OH=10 × 10 6 molecules cm −3 h) during the experiment, based on concentrations measured inside the chamber ( Fig. 5 ). The branching ratio r between the RO 2 /HO 2 reactions with NO versus other with peroxides ( Fig. 5a ) is determined using where k 3 is the reaction rate constant between HO 2 and CH 3 O 2 (7.7 × 10 −12 cm 3 molecule −1 s −1 ) at 298 K. We assume that the concentration of HO 2 and RO 2 is the same. Figure 5a illustrates that the NO pathway is dominant, by at least a factor of 20 until OH=10 × 10 6 molecules cm −3 h, and by initially thousands of times higher, over the peroxide pathway. Since r >>1 we consider these experiments ‘high NO X ’. An estimation of r during the tests on driving cycle emissions is complicated by the lack of an accurate NO X instrument (that is, one equipped with a blue light converter). Furthermore, NO was only continuously added during the experiment where emissions were sampled from the cold phase (which featured the highest VOC:NO X ratio of any experiment). However, given that the driving cycle tests generally produced higher NO emissions than the idling tests, and given that most fall on the yield curve in Fig. 2 , we also assume r >>1, although we can not rule out that during some experiments the conditions change from high to low NO X . Although the VOC:NO X ratios were high (around 50), our best estimate suggests that idling experiments were high NO X throughout. Figure 5b shows the measured concentrations of NO and O 3 , during the experiment. Idling scooter experiments Emissions were introduced into the 27 m 3 Paul Scherrer Institute Teflon environmental chamber [24] . The external temperature of the scooter exhaust was monitored (Thermocouple type K, Messelemente) and after an initial warming period of several minutes (consisting of idling or applying low power) the emissions were injected only when the external exhaust temperature was stable at idle or at simulated low power. Supplementary Table 2 provides the operating conditions, smog chamber OA concentrations and aerosol EFs of this study used in Fig. 1 . OA was monitored with a high-resolution time-of-flight aerosol mass spectrometer (Aerodyne). Unity collection efficiency is assumed, since emitted particles likely consist of spherical oil-like droplets with low bounce. After an initial spike in the OA concentration following sample injection, a time of at least 20 min was allowed for equilibration. The concentration of OA after this point was taken as the initial POA emission. A battery of 80 × 100 W ultraviolet black lights (ErgoLine ‘Cleo Performance’, Solarium lights), was used to initiate photo-oxidation and SOA formation. Experiments were carried out with a steady injection of NO (<20 ml min −1 ) whereby NO was maintained at around 2–3 ppb(v). Relative humidity inside the smog chamber was between 40–60% for all experiments, and temperature was maintained at 25 °C. OA was corrected for wall losses using where OA WLC (t) and OA MEAS (t) are the wall-loss corrected and measured organic matter concentrations, respectively, as a function of time t, and k is the first order mass-loss rate constant determined from an exponential fit of BC data. VOCs inside the smog chamber were quantified with a quadrupole proton transfer reaction mass spectrometer, while carbon monoxide was quantified with a dedicated CO monitor (Aerolaser, CO-Monitor AL5002) and total gas-phase hydrocarbons were measured from the chamber using a flame ionization detector (FID, J.U.M model VE 7). Additional measurements at the tailpipe were performed by transferring emissions through a heated line (191 °C) to a Fourier transformed infrared spectrometer (MKS Multigas analyser 2030) for online measurements (at 1 Hz) of small hydrocarbons, nitrogen containing species (NO, NO 2 , N 2 O, NH 3 and HCN) and other oxygenated small organics (formaldehyde, acetaldehyde), as well as CO and CO 2 . Online reactive oxygen species measurements Online particle-bound ROS analysis utilized the fluorescence probe 2,7-dichlorofluorescein in solution. Particles were collected and continuously extracted on a wetted hydrophilic filter. The particle collector samples air at 5 l min −1 and collects particles larger than aerodynamic diameter 50 nm with greater than 95% efficiency. Particles are collected and extracted in an aqueous solution of horseradish peroxidase (0.5 U ml −1 ) allowing immediate reaction of ROS on collection. The concentration of ROS is characterized following subsequent reaction of the oxidized horseradish peroxidase with 2,7-dichlorofluorescein (5 μM) for 10 min at 40 °C, yielding the fluorescent product DCF in the continuous flow set up. The concentration of 2,7-dichlorofluorescein is measured using fluorescence spectroscopy in a flow-through cell and calibrated to ROS concentration with hydrogen peroxide. ROS data in Fig. 3 are normalized to the total carbon m −3 , determined from high-resolution fitting of aerosol mass spectrometer data, and presented as a percentage. Driving cycle scooter experiments The Paul Scherrer Institute mobile smog chamber [3] was deployed, and experiments conducted in a certified chassis dynamometer test cell (Vehicle Emissions Laboratories, Joint Research Centre of the European Commission, JRC-Ispra, Italy) [28] , [29] . Emissions from 2S scooters were sampled at the tailpipe during full ECE47 driving cycles, during Ph1 only of the ECE47 (first four modules of the driving cycle, Ph1), and during Ph2 only of the ECE47 (final four modules of the driving cycle, Ph2). The emissions were transferred to the smog chamber via a heated inlet system (150 °C) and Dekati ejector dilutor. Ultraviolet lights were switched on after several minutes to initiate photochemistry. OA concentrations were measured with a high-resolution time-of-flight aerosol mass spectrometer (Aerodyne), while black carbon was quantified with an aethalometer (AE33, Aerosol d.o.o.). The exponential decay rate of black carbon k was used in equation (5) to correct for particle losses to the walls. Gas-phase compounds were monitored with a proton transfer reaction time-of-flight mass spectrometer (Ionicon), while CO 2 and CO were measured using a cavity ring down spectrometer (Picarro, G2401) and total hydrocarbons were measured with a flame ionization detector (Horiba, THC Monitor APHA-370). Emission factor determination EFs from both measurement campaigns (EF, g C kg −1 fuel), (see also Supplementary Table 3 ), were calculated using a carbon mass balance: where C denotes carbon mass, and the subscripts CO 2 , CO, HC, carbon dioxide, carbon monoxide and hydrocarbon, respectively. W c is the fuel carbon content (0.847 for gasoline). For the idling scooter experiments, C CO and C CO2 were measured at the tailpipe using the Fourier transformed infrared spectrometer. C HC was measured from the smog chamber and scaled-up to the tailpipe concentration using the dilution ratio CO tailpipe /CO smog chamber . Meanwhile, for the driving cycles all concentrations were determined at the smog chamber. Emission factors from the literature Figure 1 and Supplementary Table 3 show EFs calculated from the literature. When available, EFs are given as reported. OA EFs measured in tunnels/roadside are assumed to consist purely of POA and are converted to EFs in units of g kg −1 fuel using an organic matter to organic carbon ratio (OM:OC) of 1.2 (ref. 30 ). EFs given in units of g km −1 are converted using the following fuel consumptions (km kg −1 ): Asia LDVs: 16.43; US LDVs: 14.93; EU LDVs: 18.20; Heavy-duty vehicles: 2.85. EFs measured during the Kansas City vehicle study are estimated by inserting per km EFs into equation (6). SOA in Supplementary Table 3 (g C kg −1 fuel) is converted from units of g kg −1 fuel using an OM:OC ratio of 2.0 (ref. 30 ). SOA formation from 2S scooters is not available in the literature, but was estimated from emissions of aromatic hydrocarbons using a yield (see Supplementary Note 1 and Fig. 2 ) of 8.4% (suspended OA concentration 50 μg m −3 ). Further notes to individual studies are also provided in Supplementary Table 3 . How to cite this article: Platt, S. M. et al. Two-stroke scooters are a dominant source of air pollution in many cities. Nat. Commun. 5:3749 doi: 10.1038/ncomms4749 (2014).